Highly efficient inverted polymer light-emitting diodes using surface modifications of ZnO layer Organic light-emitting diodes have been recently focused for flexible display and solid-state lighting applications and so much effort has been devoted to achieve highly efficient organic light-emitting diodes. Here, we improve the efficiency of inverted polymer light-emitting diodes by introducing a spontaneously formed ripple-shaped nanostructure of ZnO and applying an amine-based polar solvent treatment to the nanostructure of ZnO. The nanostructure of the ZnO layer improves the extraction of the waveguide modes inside the device structure, and a 2-ME+EA interlayer enhances the electron injection and hole blocking in addition to reducing exciton quenching between the polar-solvent-treated ZnO and the emissive layer. Therefore, our optimized inverted polymer light-emitting diodes have a luminous efficiency of 61.6 cd A −1 and an external quantum efficiency of 17.8%, which are the highest efficiency values among polymer-based fluorescent light-emitting diodes that contain a single emissive layer. Organic/polymer-based light-emitting diodes (OLEDs/PLEDs) have been extensively used over the past few decades for display and solid-state lighting applications because of their low cost, light weight, fast response time, large viewing angle and mechanical flexibility [1] , [2] , [3] . Nevertheless, the current state-of-the-art PLEDs still have considerable room for improvement in the device efficiency and stability needed for commercial applications. To achieve OLEDs/PLEDs of high external quantum efficiency (EQE), two key parameters are important: a high internal quantum efficiency (IQE) including a high photoluminescence quantum efficiency (PLQE, η PL ) of the emissive material, singlet formation ( η s ) via spin statics and a high fraction of recombination ( η re ) of electrons and holes in the emissive layer; and a high out-coupling efficiency ( η e ) such that a high fraction of photons escape the device. In conventionally-structured PLEDs, η e is particularly poor at approximately 20% because the light generated in the emissive semiconductor is trapped and waveguided inside the OLEDs/PLEDs [4] , [5] , [6] , [7] , [8] . Inverted-structured polymer light-emitting diodes (iPLEDs) have recently been established as a the substitute for conventional PLEDs because of the good air-stability of such devices, which use high-work-function metal for the anode and air-stable metal-oxide layers for the electron- and hole-injection layers [9] , [10] , [11] , [12] , [13] . However, there are certain critical obstacles impeding the realization of highly efficient iPLEDs. In particular, the majority of the light generated in the polymeric emissive layer is fully reflected and trapped by in-plane waveguide (WG) optical modes because of the use of high-reflective-index layers such as metal-oxide ( n MO ~1.8–2.4) as the electron-injection layer, which results in low η e values for iPLEDs [14] , [15] , [16] , [17] . Thus far, several approaches have been proposed to solve the problem of waveguiding in OLEDs/PLEDs. One method of enhancing the out-coupling efficiency is to use a high-refractive-index glass substrate and a hemisphere microlens thereon [16] , [17] , [18] . Moreover, a Bragg diffraction grating (BDG), a low-index grid and an internal scattering structure of the organic layer have been introduced in these devices for the light extraction of the indium tin oxide (ITO)/organic WG mode [19] , [20] , [21] , [22] , [23] , [24] . However, BDGs fabricated using the electron-beam lithography [19] , nanoimprinting [20] and holographic methods [21] , [22] , [23] incur the high costs and require complex techniques. In addition, it is difficult to extract at broad range of light emission using BDGs with regular periodic structures for white OLEDs because such a BDG extracts specific emission wavelengths in accordance with Bragg’s law, depending on the specific grating period and angle. Even though several methods have been suggested to efficiently extract the ITO/organic and glass/air WG modes, alternative methods are still required to achieve low costs, and simple manufacturing process and efficient light extraction for a broad range of wavelengths. An additional challenge facing the development of iPLEDs is that a balance between the charge-carrier injection and transport from each electrode is crucial to increasing the efficiency of iPLEDs by improving the recombination of electrons and holes in the emissive layer. However, the charge injection and transport are unbalanced in iPLEDs that use ITO or fluorine-doped tin oxide (FTO) as the cathode; n-type metal oxide, such as zinc oxide (ZnO), hafnium oxide (HfO 2 ) or zirconium oxide (ZrO 2 ), as the electron-injection/transport layer; poly(9,9′-dioctylfluorene-co-benzo-thiadiazole) (F8BT) or poly(phenylvinylene): super yellow as the emissive layer; molybdenum oxide (MoO 3 ) or nickel oxide (NiO) as hole injection/transport layer and gold (Au) as the anode. In fact, the hole injection in this type of device indicates an ohmic contact from the MoO 3 /Au to the highest occupied molecular orbital level of the emissive layer [25] , [26] , whereas the electron-injection rates are fairly low because of the considerable energy barrier difference between the conduction band (CB) of the n-type metal oxides and the lowest unoccupied molecular orbital (LUMO) of the emissive layer [9] , [10] , [11] , [12] , [13] , [14] , [15] , [16] , [17] , [27] , [28] , [29] , [30] . Recently, various strategies have been applied to promote electron injection and transport by controlling the interface between the CB of the n-type metal oxide and the LUMO of the emissive layer by using an interlayer, such as ionic liquid molecules (ILMs) [27] , conjugated polyelectrolyte [28] , [29] , self-assembled dipole monolayer [15] , caesium carbonate (Cs 2 CO 3 ) (ref. 13 ) or barium hydroxide (Ba(OH) 2 ) (ref. 16 ). Here we show highly efficient iPLEDs by introducing a spontaneously formed ripple-shaped nanostructure of ZnO (ZnO-R) and applying an amine-based polar solvent treatment using 2-methoxyethanol (2-ME) and ethanolamine (EA) co-solvents (2-ME+EA) to the ZnO-R. In particular, we solve the critical problems facing iPLEDs by enhancing the light extraction of the WG mode using spontaneously modified ZnO-R, by improving the recombination of balanced charges via the promotion of electron-injection and hole-blocking behaviour and by reducing exciton quenching through the application of a 2-ME+EA polar solvent treatment to the ZnO-R for the ultimate iPLED devices. 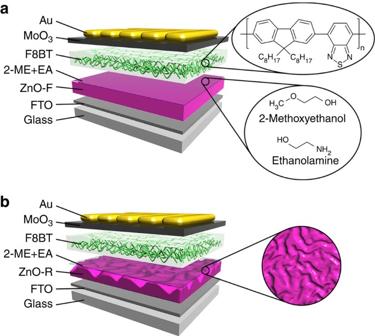Figure 1: Schematic illustrations of iPLED devices. The insets illustrate the chemical structures of the emissive layer, F8BT, and the interfacial layer, 2-ME+EA, as well as the detailed surface structure of ZnO-R. (a,b) Device architectures of iPLEDs with (a) ZnO-F and (b) ZnO-R. iPLEDs structure Figure 1a,b provide illustrations of the entire device structure of the iPLEDs, including the interfacial layer and the different surfaces of the ZnO layers: flat ZnO (ZnO-F) and ZnO-R, respectively. The insets illustrate the chemical structures of the emissive polymer, F8BT, and the interfacial layer of 2-ME and EA. The iPLEDs were fabricated via the sequential deposition of ZnO, 2-ME+EA, F8BT, MoO 3 and Au onto an FTO-coated glass substrate; this process is described in detail in the Methods section. Although the glass WG mode remains inside the device and therefore cannot contribute to the total light extraction, the ZnO/organic WG modes can be stimulated to be out-coupled by the ZnO-R. Figure 1: Schematic illustrations of iPLED devices. The insets illustrate the chemical structures of the emissive layer, F8BT, and the interfacial layer, 2-ME+EA, as well as the detailed surface structure of ZnO-R. ( a , b ) Device architectures of iPLEDs with ( a ) ZnO-F and ( b ) ZnO-R. Full size image Ripple-shaped nanostructure of ZnO The different surface properties of each type of ZnO, such as morphology, height, period and roughness, are determined by controlling the heating rate during annealing and the concentration of the ZnO solution [31] , [32] , [33] . The ZnO ripple-shaped nanostructure was formed by the reorganization of gel particles of zinc acetate dihydrate [Zn(CH 3 COO) 2 2H 2 O] during the slow drying process [34] , [35] . ZnO layers with a ripple-shaped nanostructure of lesser height and narrower width (ZnO-R1) were developed when the spin-coated ZnO samples were heated to 400 °C at a rapid heating rate (20 °C per minute), whereas structures of higher height and broader width (ZnO-R2) were fabricated using a slower heating rate (10 °C per minute). The preparation of the 2-ME+EA interlayer and the ZnO layers is described in the Methods section. Three different types of ZnO, ZnO-F, ZnO-R1 and ZnO-R2, with and without the 2-ME+EA interfacial layer were fabricated spontaneously by following the solution process using various heating rates during annealing, and the different ZnO types were confirmed via atomic force microscopy (AFM) in tapping mode, as shown in Fig. 2a–d . The ZnO-F without 2-ME+EA has a root-mean-square (rms) roughness ( R rms ) of 2.13 nm, whereas the ZnO-F with 2-ME+EA has a smoother surface with an R rms of 1.21 nm. In contrast, the ZnO-R1 with 2-ME+EA has an R rms of 3.11 nm, a height of ~30 nm and a period of ~300 nm (the dominant period over a broad wavelength range), and the ZnO-R2 with 2-ME+EA has an R rms of 13.1 nm, a height of ~70 nm, and a period of ~600 nm (the dominant period over a broad wavelength range). The periodicity of the ripple-shaped nanostructure of the ZnO layer was analysed by using the fast Fourier transform (FFT) method. Both ZnO-F layers regardless of the 2-ME+EA layer have no characteristic FFT patterns, indicating the absence of any periodic structure. In the case of the ZnO-R1 and ZnO-R2 with the interfacial layer, their FFT results exhibit ring-like patterns that represent a ripple structure with a random orientation and a spatial period. Furthermore, the power spectral density calculated from the FFT indicates that there is a significant difference in the periodicities of the ripple structures of ZnO-R1 and ZnO-R2 with a wide distribution, as shown in Fig. 2f , while no characteristic periodicity is observed in the ZnO-F layer, as shown in Fig. 2e . A spontaneously formed, randomly oriented ZnO-R layer with a wide period distribution can potentially be used as the out-coupler for the WG light to extract a broad range of emission wavelengths, regardless of direction. 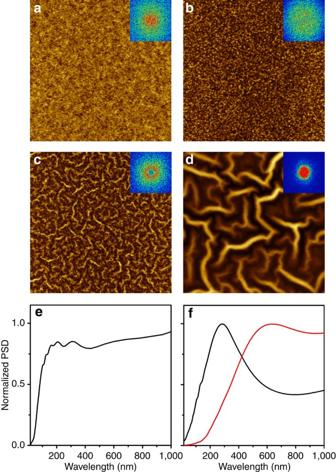Figure 2: AFM analysis of ZnO layers. Dimensions: 5 μm × 5 μm. (a–d) AFM images andRrmsvalues of ZnO-F layers (a) without (Rrms=2.13 nm) and (b) with the 2-ME+EA interlayer (Rrms=1.21 nm) and of (c) ZnO-R1 (Rrms=3.11 nm) and (d) ZnO-R2 layers with the 2-ME+EA interlayer (Rrms=13.1 nm). Insets: The FFT of each ZnO layer. Isotropic PSD plots from FFT analysis for (e) ZnO-F layers without the 2-ME+EA interlayer and (f) ZnO-R1 (black) and ZnO-R2 (red) layers with the 2-ME+EA interlayer. Figure 2: AFM analysis of ZnO layers. Dimensions: 5 μm × 5 μm. ( a – d ) AFM images and R rms values of ZnO-F layers ( a ) without ( R rms =2.13 nm) and ( b ) with the 2-ME+EA interlayer ( R rms =1.21 nm) and of ( c ) ZnO-R1 ( R rms =3.11 nm) and ( d ) ZnO-R2 layers with the 2-ME+EA interlayer ( R rms =13.1 nm). Insets: The FFT of each ZnO layer. Isotropic PSD plots from FFT analysis for ( e ) ZnO-F layers without the 2-ME+EA interlayer and ( f ) ZnO-R1 (black) and ZnO-R2 (red) layers with the 2-ME+EA interlayer. Full size image iPLED performance The device characterisations of the iPLEDs with differently structured ZnO layers (ZnO-F, ZnO-R1 and ZnO-R2) and interfacial layers are presented in Fig. 3 and Table 1 ; the presented data include (a) current density versus voltage ( J–V ), (b) luminance versus applied voltage ( L–V ), (c) luminous efficiency versus current density ( LE–J ), (d) power efficiency versus current density ( PE–J ), (e) EQE versus current density ( EQE–J ) and (f) normalized electroluminescence (EL) spectra. The efficiencies of the iPLEDs for the three different types of ZnO layers include LE s of 11.7 (ZnO-F/2-ME+EA), 14.8 (ZnO-R1/2-ME+EA) and 12.5 cd A −1 (ZnO-R2/2-ME+EA), PE s of 4.49, 5.81 and 4.93 lm W −1 , and EQE s of 3.45, 4.36 and 3.68%, respectively. In particular, the device efficiencies with ZnO-R1/2-ME+EA are higher than those for ZnO-F/2-ME+EA by approximately 25% for LE , 30% for PE and 25% for EQE because ZnO-R1/2-ME+EA can extract the ZnO/organic WG mode from inside the device structure ( Supplementary Fig. 1 ). To confirm the enhancement of the out-coupling efficiency achieved using ZnO-R, an angular-dependence measurement was conducted using an angular stage to measure the normalized EL spectra at various angles from 0° to 80°. In this study, strongly waveguided edge emission, which can occur at around 90° in the iPLEDs using high refractive index of ZnO-F, is ignored because this edge emission is useless for display applications. Interestingly, all emission patterns of the iPLEDs with ZnO-F, ZnO-R1 and ZnO-R2 are similar to that of a Lambertian pattern and the integrated EL intensities are enhanced by approximately 26% (ZnO-R1) and 11% (ZnO-R2) with respect to that of iPLED using ZnO-F (reference) because of the out-coupling effect. The use of high-reflective-index layer for the ZnO layer confines the WG modes within the interface of the ZnO and the emissive layers and the introduction of ZnO-R improves the out-coupling of the light trapped within the devices and reduces in-plane WG losses. In particular, the efficiency of the iPLED with ZnO-R2 is lower than that of the iPLED with ZnO-R1 because of the optical quenching and trapping of photons caused by the higher surface roughness of ZnO-R2. 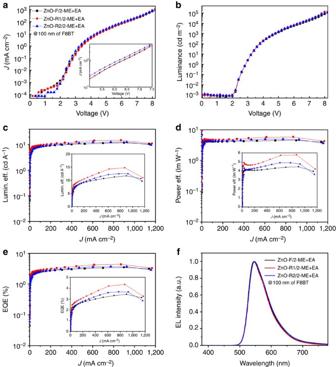Figure 3: Performances of iPLEDs with 2-ME+EA and differently structured ZnO layers. (a) Current density versus voltage (J–V) characteristics, (b) luminance versus applied voltage (L–V, cd m−2), (c) luminous efficiency (lumin. eff.) versus current density (LE–J, cd A−1), (d) power efficiency versus current density (PE–J, lm W−1), (e) EQE versus current density (EQE–J, %) and (f) normalized electroluminescence (EL) spectra of the iPLEDs. The insets ofc–eshowLE–J,PE–JandEQE–Jon a linear-linear scale. Figure 3: Performances of iPLEDs with 2-ME+EA and differently structured ZnO layers. ( a ) Current density versus voltage ( J–V ) characteristics, ( b ) luminance versus applied voltage ( L–V , cd m −2 ), ( c ) luminous efficiency (lumin. eff.) versus current density ( LE–J , cd A −1 ), ( d ) power efficiency versus current density ( PE–J , lm W −1 ), ( e ) EQE versus current density ( EQE–J , %) and ( f ) normalized electroluminescence (EL) spectra of the iPLEDs. The insets of c – e show LE–J , PE–J and EQE–J on a linear-linear scale. Full size image Table 1 Summary of device performance for iPLEDs with 2-ME+EA and differently structured ZnO layers. Full size table The efficiency of iPLEDs with ZnO-R was further increased by the application of an amine-based solvent treatment to the ZnO-R. We have demonstrated that applying a polar solvent treatment to the ZnO surface reduces the contact barrier between the active polymer and the ZnO layer because of the interfacial negative dipole effect, which is created spontaneously by the absorption of the amine (NH 2 ) and hydroxyl (OH) groups of EA on ZnO-R, enhancing the electron extraction by suppression of recombination of the electron and hole carriers [31] . The interfacial negative dipolar polarization that the nitrogen atoms and OH groups with higher electron-negativity existed near the ZnO-R surface while aliphatic groups (-CH 2 CH 2 -) with lower electron-negativity existed upward was confirmed by X-ray photoelectron spectroscopy, contact angle and ultraviolet photoelectron spectroscopy measurement. More detailed contents regarding the surface electronic structure by 2-ME+EA treatment are shown inref. [31] . To support the reduction of the electron-injection barrier between the active polymer layer and the ZnO layer and the promotion of electron injection and transport by the interfacial negative dipole effect, the current densities of the electron-only devices (FTO/ZnO-R1/F8BT/LiF/Al) with and without 2-ME+EA were measured ( Supplementary Fig. 2 ). The current density of electron-only device with 2-ME+EA is much larger than that of reference device without 2-ME+EA. This result clearly demonstrates that the electron injection and transport in the devices treated with 2-ME+EA are enhanced due to the negative dipolar polarization effect. The iPLEDs with 2-ME+EA exhibit low current densities ( J ) because of a reduced leakage current and significantly enhanced device efficiencies because of the enhanced recombination of electrons and holes inside the emissive layer (see Supplementary Fig. 4a ). Thus, the iPLEDs with ZnO-R1 and 2-ME+EA has a high luminance of 100,500 cd m −2 , an LE of 17.3 cd A −1 , a PE of 6.60 lm W −1 and an EQE of 4.91%, which are approximately 11-fold, 14-fold, 16-fold and 14-fold higher, respectively, than the corresponding values for the iPLED with the same ZnO structure without 2-ME+EA, as shown in Supplementary Fig. 4 and Supplementary Table 1 . 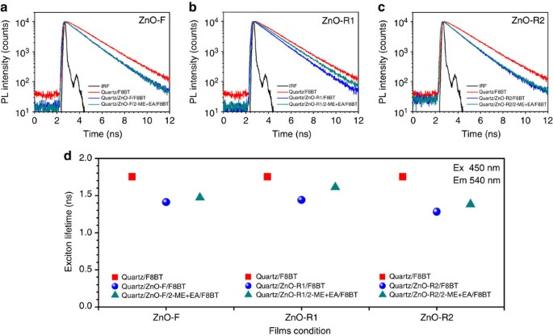Figure 4: Exciton lifetime. (a–c) Time-resolved PL signal of (a) Quartz/ZnO-F/F8BT, (b) Quartz/ZnO-R1/F8BT and (c) Quartz/ZnO-R2/F8BT with and without 2-ME+EA, measured via TCSPC at an excitation wavelength of 450 nm and an emission wavelength of 540 nm. (d) Summary of the exciton lifetimes of F8BT on the different ZnO layers. Figure 4 provides the exciton lifetimes of F8BT on various ZnO layers with and without the 2-ME+EA layer determined via time-correlated single photon counting (TCSPC). The exciton lifetimes of F8BT on ZnO-F, ZnO-R1 and ZnO-R2 are 1.44, 1.41 and 1.28 ns at 540 nm, respectively. The exciton lifetime of F8BT on ZnO-R2 is significantly shorter than that on ZnO-F because of the high surface roughness, which causes considerable exciton quenching. However, the exciton lifetime of F8BT on ZnO-R1 is comparable to that on ZnO-F. Moreover, the exciton lifetimes are increased by coating a 2-ME+EA interlayer onto the ZnO layer, which is the opposite of the results obtained when measuring exciton lifetimes for conjugated polyelectrolyte and Cs 2 CO 3 interlayers on ZnO [16] , [28] ; the application of the 2-ME+EA polar solvent treatment to the ZnO layers results in reduced exciton quenching. These results are summarized in Supplementary Table 3 . Moreover, the photoluminescence (PL) spectra of ZnO/F8BT and ZnO/2-ME+EA/F8BT were measured to support the reduction of exciton quenching by 2-ME+EA. The PL intensities of ZnO-F and ZnO-R1 with 2-ME+EA are higher than those of ZnO-F and ZnO-R1 without 2-ME+EA ( Supplementary Fig. 3 ). These PL results are in agreement with the TCSPC data, which can support the reduced exciton quenching. Therefore, it is concluded that the application of a 2-ME+EA interlayer on ZnO is effective for enhancing the electrical and optical properties of iPLED devices, as indicated by the J–V–L characteristic curves and the TCSPC and PLQE data. Figure 4: Exciton lifetime. ( a – c ) Time-resolved PL signal of ( a ) Quartz/ZnO-F/F8BT, ( b ) Quartz/ZnO-R1/F8BT and ( c ) Quartz/ZnO-R2/F8BT with and without 2-ME+EA, measured via TCSPC at an excitation wavelength of 450 nm and an emission wavelength of 540 nm. ( d ) Summary of the exciton lifetimes of F8BT on the different ZnO layers. Full size image Friend et al. [2] have previously reported that because of the large recombination zone, optimized iPLEDs can be made to exhibit LEs of more than 20 cd A −1 by controlling the width of the recombination zone with an approximately 1-μm-thick F8BT layer [16] , [36] . Here, we optimized the efficiencies of the iPLEDs by using emissive layer of different thicknesses ranging from 100 to 1,200 nm and ZnO-R1 to which the 2-ME+EA co-solvent treatment had been applied. As the thickness of the F8BT emissive layers was increased, the LE , PE and EQE improved although the luminance decreased. Among the tested devices, the iPLED with 1,200-nm-thick F8BT exhibits the highest values, with a luminance of 53,400 cd m −2 , an LE of 61.6 cd A −1 , a PE of 19.4 lm W −1 and an EQE of 17.8%, as shown in Fig. 5 and Table 2 . The device efficiencies with 1,200-nm-thick F8BT and ZnO-R1 treated 2-ME+EA are much higher than those with 1,200-nm-thick F8BT and ZnO-F treated 2-ME+EA ( Supplementary Fig. 5 and Supplementary Table 2 ). It should be highlighted that the EQE value of approximately 18% is the record high value thus far presented for fluorescent PLED devices that contain a single polymer emissive layer ( Supplementary Table 4 ). Moreover, a further increase in device efficiency can be obtained using a high-refractive-index glass substrate and a hemisphere microlens thereon to extract the glass/air WG mode, although they were not used in this study. 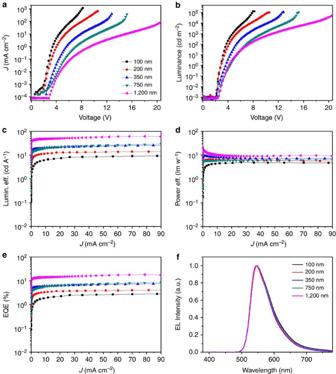Figure 5: Performance of iPLEDs devices using 2-ME+EA and ZnO-R1 with various thicknesses of F8BT. (a) Current density versus voltage (J–V) characteristics, (b) luminance versus applied voltage (L–V, cd m−2), (c) luminous efficiency (lumin. eff.) versus current density (LE–J, cd A−1), (d) power efficiency versus current density (PE–J, lm W−1), (e) EQE versus current density (EQE–J, %) and (f) normalized electroluminescence (EL) spectra of the iPLEDs. Figure 5: Performance of iPLEDs devices using 2-ME+EA and ZnO-R1 with various thicknesses of F8BT. ( a ) Current density versus voltage ( J–V ) characteristics, ( b ) luminance versus applied voltage ( L–V , cd m −2 ), ( c ) luminous efficiency (lumin. eff.) versus current density ( LE–J , cd A −1 ), ( d ) power efficiency versus current density ( PE–J , lm W −1 ), ( e ) EQE versus current density ( EQE–J , %) and ( f ) normalized electroluminescence (EL) spectra of the iPLEDs. Full size image Table 2 Summary of device performance for iPLEDs with ZnO-R1, 2-ME+EA and various thicknesses of F8BT. Full size table If we assume that the recombination ( η re ) of electrons and holes in the emissive layer is 100%, the singlet formation ( η s ) via spin statics is 25%, the PLQE ( η PL ) of the material is 100% and the light extraction ( η e ) of the iPLEDs is 25%, then the calculation indicates that a maximum EQE ( EQE = η re η s η PL η e ) of 5% can be achieved, which is significantly lower than the maximum EQE of 17.8% observed in this experiment. Two possible explanations for such a high EQE are as follows: (i) the value of η s attributable to electrical injection may be higher than 25% because of the triplet-triplet annihilation process [37] , [38] and the fact that the singlet-formation cross-section of F8BT is greater than the triplet-formation cross-section of F8BT [39] and (ii) the enhanced light extraction ( η e ) of the iPLEDs achieved by using ZnO-R may also contribute to the high EQE value. Finite-difference time-domain calculation To investigate the enhanced device performance with regard to light extraction, we calculated the dispersion curves of the proposed OLED devices. We used the finite-difference time-domain method to enable the calculation of the dispersion curves of the nanostructure-incorporated devices. In this calculation, we compared the flat device (ZnO-F) to the nanostructured device (ZnO-R1) by assuming a uniform shape (hemi-ellipse) and pattern space (Λ=300 nm) of the ZnO nanostructures to simplify the random nature of the nanopatterns. Supplementary Figure 6 provides the calculated dispersion curves for the transverse-magnetic and transverse-electric modes of the ZnO-F and ZnO-R1 devices. Supplementary Figure 6b,d clearly indicate the extraction of guided modes into the air cone when the corrugated nanostructures are incorporated, but no such extraction is evident in the case of the flat device ( Supplementary Fig. 6a,c ). Even though the exact theoretical calculation of the extraction efficiency is not available due to the random nature of the patterns and the limitation of two-dimensional simulation, the extraction efficiency and the optical loss of the iPLEDs was obtained by integrating the corresponding region in the power dissipation spectrum shown in Supplementary Fig. 6 (ref. 40 ). In the case of ZnO-F and ZnO-R1 devices, the amount of power emitted directly to air ( k x < k n_ air=1 ) is increased from 19 to 34% and the optical loss including waveguided and SPP modes ( k x >k n_ glass=1.52 ) is decreased from 35 to 26%. It implies that the enhancement of extraction efficiency is about 79% for the iPLED with ZnO-R1 compared with ZnO-F. We believe that the extraction is primarily attributable to the reduction in the in-plane wave vectors of the WG modes caused by the Bragg grating vector [7] , [8] . To clarify the higher extraction in the ZnO-R1 device (Λ=300 nm) compared with that in the ZnO-R2 device (Λ=600 nm), we calculated the grating period as a function of the emission wavelength, as shown in Supplementary Fig. 6e (ref. 7 , 8 ). It should be noted that the corrugation period of the ZnO-R1 device (Λ=300 nm) is well matched with the grating period that is required to extract the WG modes for the emission wavelength (~540 nm). These simulated results are consistent with the experimental observations ( Fig. 3 , Supplementary Fig. 1 ). In this article, we successfully achieve an ultimate LE of 61.6 cd A −1 , a PE of 19.4 lm W −1 and an EQE of 17.8% in iPLEDs using a simple and effective method that relies on the nanostructure of ZnO-R and the 2-ME+EA polar solvent treatment of the ZnO-R. Spontaneously formed ZnO-R effectively enhances the extraction of the ZnO/organic mode, and this enhancement is independent of the specific grating period and polar angle because of the broad periodicity distribution and the random orientation. Moreover, modification of the interface using 2-ME+EA controls the energy barrier between the CB of the ZnO-R and the LUMO of the emissive layer to balance the injection of charges, which results in highly efficient iPLEDs. Furthermore, our approach can be applied to white PLEDs and electrically pumped organic lasers. ZnO-R/2-ME+EA film fabrication A 0.75-M ZnO-R solution was synthesized by dissolving zinc acetate dehydrate [Zn(CH 3 COO) 2 2H 2 O] in 2-methoxyethanol and ethanolamine co-solvents. This solution was stirred at 60 °C for 30 min to yield a clear and homogeneous solution [31] , [32] , [33] . The ZnO-R precursor solution was spin-cast onto cleaned FTO substrates after a 30-min UV-ozone treatment and heated to 400 °C with a heating rate of 20 °C per minute (ZnO-R1) or 10 °C per minute (ZnO-R2). Subsequently, the ethanolamine/2-methoxyethanol (1:20 (vol. %)) was spin-cast at 3,000 r.p.m. on top of the ZnO-R layer and then dried at 140 °C for 10 min. AFM characterization The surface roughnesses and morphologies of the ZnO-F, ZnO-R1 and ZnO-R2 films with and without the 2-ME+EA layer were measured using AFM (Veeco Co.). iPLED cell fabrication and characterization FTO substrates were cleaned in an ultrasonic bath using a conventional cleaning process with deionised water (DI water), acetone and isopropyl alcohol and were then dried under a stream of N 2 . The ZnO layers were spin-coated onto FTO substrates after a 30-min UV-ozone treatment and were then heated to 400 °C with different heating rates. Then, the 2-ME+EA co-solvent was spin-cast on top of the ZnO layers and dried at 140 °C for 10 min under ambient atmosphere. The emissive layer of F8BT (Cambridge Display Technology Ltd. (Mn=114 kg mol −1 ) was spin-coated from a p -xylene solution onto the prepared ZnO-R/2-ME+EA film and then annealed at 155 °C for 1 h under nitrogen. A MoO 3 (10 nm) and Au (100 nm) electrode were deposited via thermal evaporation under vacuum conditions (<10 −6 Torr). The area of the device was 13.0 mm 2 . The J–V–L characteristics and efficiencies were measured using a Keithley 2400 Source Meter and a Konica Minolta spectroradiometer (CS-2000), respectively. Time-correlated single photon counting The exciton lifetime was measured by using the TCSPC method. The details are shown in ref 41 . How to cite this article: Lee, B. R. et al. Highly efficient inverted polymer light-emitting diodes using surface modifications of ZnO layer. Nat. Commun. 5:4840 doi: 10.1038/ncomms5840 (2014).